Graphene etching on SiC grains as a path to interstellar polycyclic aromatic hydrocarbons formation Polycyclic aromatic hydrocarbons as well as other organic molecules appear among the most abundant observed species in interstellar space and are key molecules to understanding the prebiotic roots of life. However, their existence and abundance in space remain a puzzle. Here we present a new top-down route to form polycyclic aromatic hydrocarbons in large quantities in space. We show that aromatic species can be efficiently formed on the graphitized surface of the abundant silicon carbide stardust on exposure to atomic hydrogen under pressure and temperature conditions analogous to those of the interstellar medium. To this aim, we mimic the circumstellar environment using ultra-high vacuum chambers and investigate the SiC surface by in situ advanced characterization techniques combined with first-principles molecular dynamics calculations. These results suggest that top-down routes are crucial to astrochemistry to explain the abundance of organic species and to uncover the origin of unidentified infrared emission features from advanced observations. The great advances experienced by radioastronomy during recent years have depicted the interstellar medium (ISM) and circumstellar envelopes (CSE) as supporting an active and rich chemistry [1] . In these cosmic regions, both simple molecules, such as H 2 or CO, and complex ones, such as C 60 and polycyclic aromatic hydrocarbons (PAHs), are routinely detected by their characteristic infrared spectrum [2] , [3] . Advances in infrared spectroscopy, powered by space missions such as ISO and Spitzer , have revealed the existence of dust grains composed of silicates, SiC or oxides, among other substances, in such regions [4] , [5] , [6] . All this chemical complexity present in the ISM and in CSEs plays a major role in the evolution of galaxies, comets, the formation of planets and, ultimately, in the abiotic organic chemistry that preceded the origin of life on Earth [7] . PAHs contain up to 20% of the carbon in the photodissociation regions [8] , and are present in any region subjected to ultraviolet radiation [9] . However, despite being so ubiquitous and playing such a crucial role in several astrophysical processes and environments, their formation in the interstellar and circumstellar media remains poorly understood. Proposed chemical routes leading to the formation of complex polyaromatic molecules, and particularly to large PAHs, in space cannot account for their abundance and thus efficient mechanisms for their formation are still an open issue. The main current theories invoke either combustion-like [10] , [11] , [12] or ultraviolet-driven—acetylenic—polymerization and evaporation processes in most evolved objects [13] , [14] , [15] , [16] , [17] . However, the efficiency of such processes is still unknown [8] , [9] , [18] and during the last 30 years an important amount of work has been performed to determine PAHs origin and physicochemical properties. Unfortunately, a complete carbon inventory is difficult to determine, as many other important molecules—such as carbon clusters (C 2 , C 3 , C n ), CH 4 and C 2 H 4 , which could also be abundant in the inner regions of CSEs—have not yet been quantitatively observed with sufficient detail. Within this context of chemical complexity in the ISM, new bottom-up assembling mechanisms based on concepts from nanotechnology have recently come into play. The catalytic role of interstellar dust grains in certain reactions has long been proposed; in their seminal work, Watson and Salpeter [19] and later Hornekaer et al. [20] studied the dust grains as the preferred sites for the formation of the most abundant molecule, H 2 . In this article, we propose—and experimentally reproduce—an alternative and efficient mechanism based on a top-down approach for producing PAHs through the hydrogen processing of SiC dust grains, which is schematically shown in Fig. 1 . Such SiC grains are formed in the inner regions (1–5 R *, R * stellar radius) of evolved stars by means of gas-phase condensation [14] , [18] . We show that in space, SiC crystallites possess a significant amount of segregated carbon on their surfaces, primarily organized as graphitic overlayers. These grains travel through the CSE owing to the radiation pressure induced by the infrared photons of the central star, until they reach the cold external layers of the envelope. At this point (>5 R *), they are exposed to ultraviolet radiation. PAH emission has been observed to be prominent in photodissociation regions where most molecules are photodissociated and dust grains are processed [2] , [8] . Here ultraviolet photons and H atoms produced by H 2 photodissociation further process the grain surfaces. We show experimentally that atomic H interaction at elevated temperature (1,000–1,300 K) on a graphene-terminated SiC surface, where graphene denotes a single layer of carbon atoms arranged in a honeycomb structure, triggers significant surface erosion even at low atomic H exposures. Thus, the graphene layer at the SiC crystallite surface is etched, leading to the formation of broken graphene flakes with sizes ranging from a few carbon rings to large graphene areas. This provides a method to inject PAHs and other PAH-related species into the gas phase. 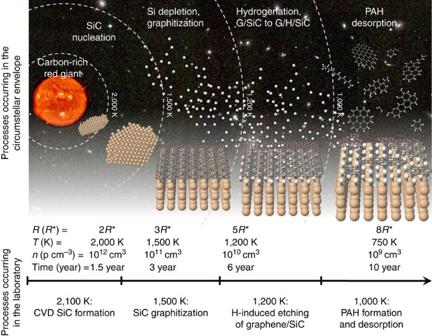Figure 1: Qualitative sketch of the proposed process. The steps for the formation of interstellar PAHs and aromatic-aliphatic molecules in the envelope of an evolved star can be divided into four different stages. (1) Formation of SiC in the gas phase and condensation into micrometre- and nanometre-sized grains (T=2,000 K; 1–5R*). (2) Annealing of the SiC dust grains due to the proximity of the star and the consequent promotion of surface C-rich phases and graphene (T=2,000–1,500 K, 1–5R*). (3) Exposure of the surface to atomic hydrogen, promoting graphitization of the C-rich surface and H passivation of the underlying buffer layer (T=1,500–1,200 K; 5–20R*). (4) Etching of the graphene by atomic hydrogen and thermally assisted desorption of PAHs (T=1,200–1,000 K, 5–20R*). Temperature values are taken from ref.36. Lower row: typical temperature in laboratory experiments. Figure 1: Qualitative sketch of the proposed process. The steps for the formation of interstellar PAHs and aromatic-aliphatic molecules in the envelope of an evolved star can be divided into four different stages. (1) Formation of SiC in the gas phase and condensation into micrometre- and nanometre-sized grains ( T =2,000 K; 1–5 R *). (2) Annealing of the SiC dust grains due to the proximity of the star and the consequent promotion of surface C-rich phases and graphene ( T =2,000–1,500 K, 1–5 R *). (3) Exposure of the surface to atomic hydrogen, promoting graphitization of the C-rich surface and H passivation of the underlying buffer layer ( T =1,500–1,200 K; 5–20 R *). (4) Etching of the graphene by atomic hydrogen and thermally assisted desorption of PAHs ( T =1,200–1,000 K, 5–20 R *). Temperature values are taken from ref. 36 . Lower row: typical temperature in laboratory experiments. Full size image The potential of surface science methodology to mimic and characterize the essential characteristics of complex problems concerning molecules on surfaces has been previously demonstrated by explaining, among others, the fundamentals of catalysis [21] or the formation of H 2 on the stardust grains [20] . We simulate the conditions of interstellar space using ultra-high vacuum (UHV) chambers equipped with in situ atom-resolved scanning tunnelling microscopy (STM) and third-generation synchrotron radiation-based X-ray photoemission-spectroscopy (XPS), among others. The experimental results are confirmed by ab initio calculations. This theory–experiment combination provides a state-of-the-art morphological, structural and spectroscopic description about molecular interactions on SiC crystallites under CSE conditions. In addition, SiC has also been widely studied in condensed matter research and nowadays it is well accepted that all SiC crystalline structures are covered with graphene after annealing in vacuum [22] , [23] . Graphitized interstellar SiC Dust grains produced in Carbon-rich asymptotic giant branch stars are abundant in SiC crystallites [18] . Their size can range from few nm in the proximities to the star to some μm. Extra-solar particles of SiC as big as 5 μm have been found in the interior of chondritic meteorites [24] , [25] . The most common circumstellar SiC polytypes, as found in the Murchison meteorite are 3C-SiC (80%) and 2H-SiC (16%). The size of the SiC grains in the ISM is sufficiently large to present atomically reconstructed facets and their main chemical aspects can therefore be confidently simulated by the use of SiC single crystals. We have used as an analogue to the dust grains a 6H-SiC(0001) single crystal, and the data were taken with a base pressure in the range of 10 −11 mbar, similar to the conditions occurring in the densest regions of the ISM [26] (see Supplementary Note 1 ). Because of temperature-induced Si sublimation and subsequent C segregation, the surface of SiC crystallites is always graphitized after annealing at typical temperatures of the ISM depletion zone ( Fig. 1 ). In the case of SiC(0001), the surface after annealing at 1,500 K consists of a combination of atomically flat terraces partially covered with single-layer graphene ( Fig. 2a ) and other areas with a carbonaceous termination consisting either of a mixture of Si and C atoms in sp 2 / sp 3 configuration or bilayer graphene (BLG) [23] , [27] . The graphene termination of different SiC specimens after being submitted to high temperature has been observed in different previous studies, both for large grains or small nanoparticles [22] , [23] . Therefore, we conclude that the SiC grains present at CSE end with a graphene cover, as the one shown in Fig. 2a . 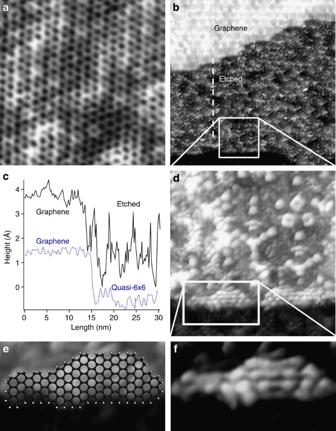Figure 2: Graphene etching on high-temperature and atomic H dose. (a) STM image (5 × 5 nm2) showing a graphene regionV=100 mV; the small mesh corresponds to the atomic honeycomb atomic lattice of graphene. (b) The image shows at the upper side a graphene plane, whereas at lower part the surface has strongly roughened. 40 × 40 nm2V=−100 mV. (c) Profile on STM images recorded before (blue) and after (black) being exposed to atomic H with the surface kept at 1,200 K, taken along the dotted line indicated in. The total roughness (r.m.s.) of the surface increases from 0.22 to 0.69 Å. (b,d–f) Series of STM images showing the graphene surface eroded after atomic H exposure at high temperature. (d) STM image (10 × 10 nm2) recorded on the most eroded part that shows the formation on the surface of small molecules and nanostructures.V=−200 mV (f) STM image (2.2 × 4 nm2) zooming in on a detail of the surface showing protrusions corresponding to localized molecular orbitals of a PAH-like molecule. (e) Overlaid optimized DFT model of a proposed PAH formed. Figure 2: Graphene etching on high-temperature and atomic H dose. ( a ) STM image (5 × 5 nm 2 ) showing a graphene region V =100 mV; the small mesh corresponds to the atomic honeycomb atomic lattice of graphene. ( b ) The image shows at the upper side a graphene plane, whereas at lower part the surface has strongly roughened. 40 × 40 nm 2 V =−100 mV. ( c ) Profile on STM images recorded before (blue) and after (black) being exposed to atomic H with the surface kept at 1,200 K, taken along the dotted line indicated in. The total roughness (r.m.s.) of the surface increases from 0.22 to 0.69 Å. ( b , d – f ) Series of STM images showing the graphene surface eroded after atomic H exposure at high temperature. ( d ) STM image (10 × 10 nm 2 ) recorded on the most eroded part that shows the formation on the surface of small molecules and nanostructures. V =−200 mV ( f ) STM image (2.2 × 4 nm 2 ) zooming in on a detail of the surface showing protrusions corresponding to localized molecular orbitals of a PAH-like molecule. ( e ) Overlaid optimized DFT model of a proposed PAH formed. Full size image G/SiC exposed to atomic hydrogen As the surface-graphitized SiC grains travel outwards into the ISM they cool (1,500–1,000 K). During this trip, they are exposed to ultraviolet-photodissociated atomic H with an approximate impinging rate of ≈1 × 10 14 particles cm −2 s. These are the conditions we use to simulate the process: a temperature of about 1,200 K while exposing the surface to an approximate dose of 4 Langmuir (L; 1 L=10 −6 mbar s≈10 15 particles cm −2 s) of atomic H. Figure 2c–e shows STM images at different length scales with atomic resolution demonstrating that the graphene-covered SiC surface has been strongly modified. The upper part of the image in Fig. 2b still contains grapheme, whereas the lower region has been completely etched and roughens. In the etched part some remaining carbonaceous pieces can be observed (brighter features in Fig. 2d ). To emphasize the erosion process, we show in Fig. 2c a height profile of an etched surface recorded on Fig. 2b after dosing the crystallite with atomic H and for comparison a height profile of an as-grown surface. The peak-to-valley difference is about 3 Å, which is the size of an atomic step in the SiC surface, suggesting that a whole layer has been disrupted. It is clear that the corrugation of the profiles strongly increases after H dosing at high temperature, indicating a strong erosion of the carbon termination. In general, on H exposure at elevated temperature, the surface tends to reorganize from sp 3 to sp 2 configuration [27] , leading to a cracked and decoupled graphene layer from the SiC surface. Figure 2d shows some formed carbonaceous structures of different sizes remaining weakly bound to the surface. High-resolution images reveal some features that can be assigned to large PAHs (see Fig. 2e,f ). These features show a molecular orbital-like electronic density and a periodicity of about 2.4 Å between bright lobes [28] . This distance corresponds to the lattice constant of graphene, indicating that these structures consist of a concatenation of benzene rings (see Supplementary Note 2 and Supplementary Figs 1 and 2 ). This situation leaves small patches of graphene weakly bound to a H-saturated substrate, ready to be ejected by thermal or photoexcitation processes. These molecules could be the origin of the recently proposed top-down interstellar carbon chemistry [29] and the reason why SiC is abundant in evolved stars but normally gone in the ISM [30] . 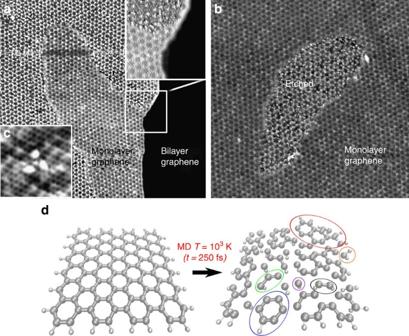Figure 3: STM images after H dosing at 1,100 K of G/SiC and computer simulation. (a) 100 × 100 nm2, −1,100 mV. Wide view of a region where the graphene has been reduced to a stripe with rounded edges on the centre of the image. On the right part of the image, a region of BLG seems unaltered. The upper inset shows a high-resolution image of a kink where single-layer graphene, BLG and the modified etched substrate coexist. (b) STM image of a hole in the middle of a graphene terrace. These holes are observed after H treatment at high temperatures and they evidence etching through edges and defects. 70 × 70 nm2, −1.1 V. (c) Atomically resolved STM image of a subsurface trimmer 2.5 × 2.5 nm2, −400 mV. (d) Initial and final frames of the graphene surface extracted from a movie of DFT molecular dynamics calculations of the G/H/SiC system. The distance between graphene layers expand from 7% at room temperature to about 62% at 1,000 K, and finally, after 250 fs (MD time), the topmost layer disrupt in the form of small carbonaceous species. In this case, benzene rings (blue oval), acetylene molecule (black oval), methylene radical (orange oval) or PAHs (red oval) can be identified. Figure 3a,b shows some regions of the surface that have been heavily etched. Figure 3a displays an area where the graphene cover has been strongly shrunk to small patches. Only graphene islands remain in the centre of the image. The most probable scenario is that the original flake covered the whole upper terrace (brighter area at the left side of Fig. 3a ) and continued over another graphene layer into the lower terrace (darker area at the right side of Fig. 3a ). The etching process has attacked the graphene in contact with the H-passivated substrate, and the process has stopped at the step edge where the overlayer becomes BLG. Thus, the presence of BLG can be considered as a protective film with respect to H attack [31] , [32] . This could be the reason why this process does not disrupt the whole SiC grain. Figure 3b shows a graphene area where a small flake has been blown out from the surface and the contour of the etched region is visible. The flakes exhibit rounded smooth contours, and high-resolution images show heavily distorted electronic states at the edges, which could originate from passivation through hydrogenation of the edge atoms [33] . In both images of Fig. 3 can be seen that the edge between graphene and eroded parts is strongly modified, indicating that H erosion takes place through edges and defects of the graphene layer. These structural defects are spots to intercalate H atoms into the graphene structure. In some parts of the surface, we have found evidences of H inserted between the SiC interface and the graphene layer. The Fig. 3c shows three bumps identified by their apparent height as H atoms adsorbed on the lower basal plane of graphene. Figure 3: STM images after H dosing at 1,100 K of G/SiC and computer simulation. ( a ) 100 × 100 nm 2 , −1,100 mV. Wide view of a region where the graphene has been reduced to a stripe with rounded edges on the centre of the image. On the right part of the image, a region of BLG seems unaltered. The upper inset shows a high-resolution image of a kink where single-layer graphene, BLG and the modified etched substrate coexist. ( b ) STM image of a hole in the middle of a graphene terrace. These holes are observed after H treatment at high temperatures and they evidence etching through edges and defects. 70 × 70 nm 2 , −1.1 V. ( c ) Atomically resolved STM image of a subsurface trimmer 2.5 × 2.5 nm 2 , −400 mV. ( d ) Initial and final frames of the graphene surface extracted from a movie of DFT molecular dynamics calculations of the G/H/SiC system. The distance between graphene layers expand from 7% at room temperature to about 62% at 1,000 K, and finally, after 250 fs (MD time), the topmost layer disrupt in the form of small carbonaceous species. In this case, benzene rings (blue oval), acetylene molecule (black oval), methylene radical (orange oval) or PAHs (red oval) can be identified. Full size image DFT and MD theoretical analysis To shed some light on the etching of the graphene by atomic hydrogen, and the subsequent thermally assisted PAH formation and desorption at T =1,000 K and beyond 5 R * (see Fig. 1 ), we have carried out density functional theory (DFT)-based atomistic molecular dynamics (MD) simulations. To fully understand the mechanism underlying the PAH formation and desorption, we have designed three heuristic theoretical procedures: first, to mimic the behaviour of BLG, we have performed MD simulations ( T =1,000 K) of two parallel 6 × 6 H-saturated graphene nanoribbons (with 132 atoms each) distanced by 3.35 Å, see Supplementary Movies 1–3 ; second, to quantify the influence of interlayered atomic hydrogen in the PAH formation and desorption process, we have repeated the MD calculations of the nanoribbon by including around 0.5 ML atomic hydrogen content in between the interlayer region, see Supplementary Movies 4–6 ; and finally, to simulate the thermally assisted behaviour of a graphene single layer, we have performed MD calculations ( T =1,000 K) of a 6 × 6 H-saturated graphene nanoribbon on a (fix) fully pre-optimized fragment of on-SiC graphene buffer layer (at a distance of 3.35 Å), with the same interlayer atomic H content than in previous case (around 0.5 ML), see Supplementary Movies 7–9 . All these molecular dynamics calculations have been carried out up to a total time of 250 fs (in steps of 1 fs) at 1,000 K. The fourth set of movies ( Supplementary Movies 10–12 ) is calculated with the same conditions than the last set; this is with a pre-optimized fragment of fixed buffer layer but the timescale is larger, up to 1,000 fs. From this exhaustive theoretical analysis, we can conclude that the highest PAH formation and desorption efficiency is observed for the graphene single layer on the fix on-SiC graphene buffer layer with a high atomic hydrogen content in between the interlayer region, as evidenced in the STM experiments. For this case, after 250 fs, MD process reveals a C–C broken bond ratio of around 60%, to be compared with the 30 and 5% for the hydrogenated and clean graphene bilayer, respectively. The lower PAH formation and desorption efficiency for the hydrogenated BLG may be explained in terms of that the two free-to-move graphene layers forming the bilayered system can structurally follow, adapt and accommodate the vibrations thermally induced in each other, reducing in this way the efficiency (with respect to the single-layer graphene). Graphene on SiC crystallites is supported on a strongly bonded (almost unaltered) buffer layer, which is unable to accommodate the thermally induced vibrations in the supported graphene single layer. Lower etching efficiency in BLG has been experimentally confirmed in Fig. 3 . Figure 3d shows the structure of the starting graphene flake on the on-SiC graphene buffer layer before (left panel, t =0), and after (right panel, t =250 fs) the MD calculation, showing the initial stages of PAH formation and desorption. The MD simulations reveal that, at T =1,000 K, the atomic hydrogen located in between the interlayer region starts to attack the already H-saturated edges of the nanoribbon, favouring the rupture of the external C–C bonds, and the creation of some CH 2 groups. As the time increases, the atomic hydrogen located in the interlayer region starts to attach to more internal C–C bonds in the ribbon, inducing their rupture, as well as the formation of CH and C 2 H 2 groups, and small aliphatic C 3 H n chains. From around 200 fs, all the functional groups tend to separate from each other and desorbs by expansion, and some larger structures can be observed, such as some aromatic rings and larger PAHs. In addition, to theoretically quantify the graphene-decoupling pattern by the intercalated hydrogen with temperature, we have performed an additional optimization calculation (at T =0 K), by including the van der Waals interaction in a perturbative way (see ref. 34 and references therein), of an infinite graphene bilayer with a 0.5-ML of intercalated atomic hydrogen content. The result of this optimization process shows the intercalated hydrogen atoms attaching to internal (basal) on-top carbon positions leading to a net interlayer distance dilatation from 3.35 Å—for the pristine bilayered graphene—to an interlayer distance of 3.60 Å—for the bilayered graphene—which can be quantified in a net graphene decoupling of 7% with respect to the clean system. This value can be easily compared with the decoupling rates extracted from the molecular dynamics simulations (at T =1,000 K) of the previously mentioned calculations (the pristine bilayered graphene and its H-intercalated form) after a molecular dynamics time of 250 fs. For these systems, the decoupling rates can be estimated to be around 19% for the pristine graphene bilayer at T =1,000 K (an average interlayer distance dilatation from 3.35 to 3.98 Å) and in around 62% for the graphene bilayer with intercalated atomic hydrogen at T =1,000 K (an average interlayer distance dilatation from 3.35 to 5.42 Å). This behaviour clearly manifests that both the temperature and the intercalated atomic hydrogen content improve the graphene-decoupling efficiency. Nevertheless, according to the previous numbers, the influence of the intercalated atomic hydrogen is substantially higher (around three times higher) than the temperature, showing its important catalytic role in this graphene-decoupling reaction. XPS C1s intensity on H exposition at high temperature The above-proposed mechanism is based on topographical information obtained from high-resolution STM images and DFT calculations. To confirm them, and to acquire quantitative information, we explore the relevant chemistry by analysing high-resolution synchrotron radiation XPS spectra before and after H exposures. The C1 s core level peak gives an indication of the atomic density of C at the surface region of a sample and the particular electronic environment (that is, bonding configuration) [35] . 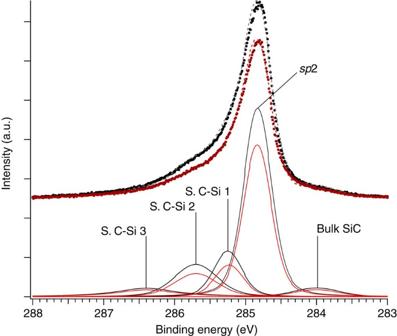Figure 4: Synchrotron-based XPS spectra of C1s. The spectra are shown before (black curve) and after (red curve) H treatment (550 L) at 1,200 K. Beneath the experimental data, we show their decomposition into separate curve components. A decrease in the C peak of about 28% in the surface-related components indicates that those C species have been etched away through H processing. The component appearing at 284.8 eV can be assigned to the graphenesp2configuration. The components located at lower binding energies (about 284.0 eV) are attributed to bulk carbides and the components at the left-hand side of the spectra to the buffer layer (between graphene and SiC). Photon energy: 400 eV. Figure 4 shows the C1s spectrum of the SiC before and after exposure to 550 l of atomic H at 1,250 K. This peak, as well as the Si2 p peak (see Supplementary Fig. 3 ), can be decomposed into different components in good agreement with the scientific literature [35] , [36] (see Supplementary Note 3 for Si2 p curve components decomposition). The component appearing at 284.8 eV can be assigned to the graphene sp 2 configuration and is the biggest contribution to the C spectra (58.2% of the total), consistent with the area estimation from the STM topography. The components located at lower binding energies (about 284.0 eV) are attributed to bulk carbides and the components at the left-hand side of the spectra to the buffer layer [35] . Figure 4 shows that the whole intensity of the C 1 s peak decreases on H exposure treatment, indicating that there is about a 30% of carbon desorption, which left the surface with lower density than the original one. Although this number cannot be directly extrapolated to the CSE, the high efficiency of the presented erosion process makes these events highly probable to occur at the CSE regions. Figure 4: Synchrotron-based XPS spectra of C1 s . The spectra are shown before (black curve) and after (red curve) H treatment (550 L) at 1,200 K. Beneath the experimental data, we show their decomposition into separate curve components. A decrease in the C peak of about 28% in the surface-related components indicates that those C species have been etched away through H processing. The component appearing at 284.8 eV can be assigned to the graphene sp 2 configuration. The components located at lower binding energies (about 284.0 eV) are attributed to bulk carbides and the components at the left-hand side of the spectra to the buffer layer (between graphene and SiC). Photon energy: 400 eV. Full size image If we perform the intensity analysis of the components of the C 1 s peak before and after H exposition, while keeping the sample at high temperatures, we can study the modification degree of every component. The C1 s core level peak and its components indicate the quantity and density of carbon present on the sample. By tracking the changes in the intensity of every component, we can follow the modification of the carbon species upon H exposition. Therefore, in case the intensity of some particular component decreases, we can assume the number of carbon atoms in such bonding configuration is diminishing. The components of the C1 s peak are divided in two ranges of modification after hydrogen treatment at high temperatures. The components at energies 284.8, 286.4 and 284.0 eV decrease, respectively, by −19.4, −19.4 and −20.7% while the components at energies 285.25 and 285.7 eV change by −30.2 and −29.8%. This evidences a loss of carbon atoms on the surface in a disordered manner that leaves the surface with a smaller C density than before the hydrogen treatment. If the carbon atoms would leave the surface in a layer-by-layer mechanism, we would find an XPS spectra modification that eventually would return the intensity and shape to its original spectra, indicating that a full layer has been eroded and a new one is exposed to the X-rays. As the C1 s peak intensity decreases only in two different values: approximately −20% for the graphene, bulk and S. C-Si 3 components, and approximately −30% for the surface S. C-Si 1 and S. C-Si 2 components, three values in the Si2 p (~13.5, ~+4 and ~20%) indicates certain relation between the components sharing the same degradation. The less altered components pertain to the most buried electronic configurations as the hydrogen will mostly attack the atoms located at the surface–vacuum interface. Therefore, the C bulk component is less altered than the surface S. C-Si 1 and S. C-Si 2 components. The exceptions are the graphene and the S. C-Si 3 components that are less altered than the other two surface components. This might arise because of a lower efficiency of the etching process at the carbon atoms in such configurations. 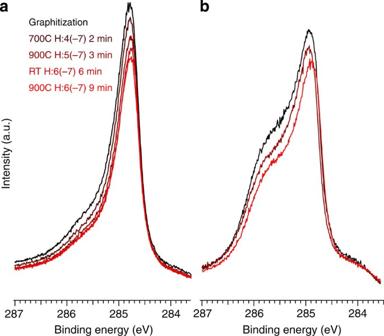Figure 5: High-resolution evolution of the XPS core level peak of C1s. (a) Spectra corresponding to the exposure of a graphene covered SiC (1 ML) surface to atomic H at different temperatures during different times. (b) Spectra corresponding to the exposure of a partially graphene-covered SiC surface, surface to atomic H at different temperatures and doses: black curve (as graphitized), brown curve (first two steps of a figure, that is, 2 min at 700 C and 4 × 10−7mbar and later 3 min at 900 C and 5 × 10−7mbar) and red curve (second two steps ofa, that is, 6 min at 30 C and 6 × 10−7mbar followed by 9 min at 900 C and 6 × 10−7mbar. The photon energy for both spectra is 400 eV. Figure 5a shows the evolution of the lineshape of the C1 s peak after subsequent different treatments involving exposition to H atmospheres at different temperatures. The original graphitization degree of the sample is around one monolayer. After a first cycle, 50 L of atomic hydrogen while keeping the sample at 1,000 K, the C1 s intensity decreased 5%. Subsequently, we exposed it to a second cycle, 90 L with a sample temperature of 1,200 K, that resulted in an extra 7% intensity loss. The third subsequent cycle was performed keeping the sample at room temperature (300 K) and submitting it to a hydrogen dose of 220 L, and it resulted in an extra intensity loss of 3%. The last cycle performed on this sample consisted of 325 L of atomic hydrogen while the sample was kept at 1,200 K, and it resulted in an extra 3% decrease of the photoelectron intensity. In total, we dosed around 685 L of hydrogen on the sample, which caused a total intensity decrease of 19%. Importantly, in all the steps of the experiment using low hydrogen pressure, the XPS intensity was reduced after high-temperature dose. This experiment is an indication of the low-pressure etching efficiency on SiC samples with graphene coverage around one monolayer. Figure 5: High-resolution evolution of the XPS core level peak of C1 s . ( a ) Spectra corresponding to the exposure of a graphene covered SiC (1 ML) surface to atomic H at different temperatures during different times. ( b ) Spectra corresponding to the exposure of a partially graphene-covered SiC surface, surface to atomic H at different temperatures and doses: black curve (as graphitized), brown curve (first two steps of a figure, that is, 2 min at 700 C and 4 × 10 −7 mbar and later 3 min at 900 C and 5 × 10 −7 mbar) and red curve (second two steps of a , that is, 6 min at 30 C and 6 × 10 −7 mbar followed by 9 min at 900 C and 6 × 10 −7 mbar. The photon energy for both spectra is 400 eV. Full size image The etching process also takes place on samples with a graphene layer covering less than one monolayer. In Fig. 5b , we see the C1 s XPS core level spectra of a SiC sample whose degree of graphitization is lower than one monolayer. The intensity after submitting the sample to cycles of hydrogen treatment at high sample temperatures (1,000–1,200 K) diminishes around 14%. The degree of modification of the hydrogen etching is dependent, in a non-trivial manner, on the hydrogen dose, the temperature of the sample during the exposition and the original degree of graphitization of the sample. Surface science aims at studying highly controlled systems and tracing the influence of particular parameters in the final product of a chemical transformation. This approach has produced outstanding results in different fields, such as solid-state chemistry or catalysis [21] . The environmental parameters in our simulation chambers, such as temperature, vacuum and gas composition, were as close as possible to the conditions occurring in the CSE. Of course, real CSEs have a much complex chemistry than the one gathered in our experimental ideal environmental simulation chambers. Molecules such as H 2 , CO or C 2 H 2 are present in the proximities of evolved carbon-rich stars [37] , and electromagnetic radiations, covering large regions of the spectrum, have non-negligible intensities in the vicinities of the stars. These parameters might play a role in the mechanism proposed here for the formation of PAHs. However, in the case of the mechanism that we are proposing, the role of radiation and small molecules is not so important. First, because graphene absorbs electromagnetic radiation through excitation of vibrational phonon modes, which later decay through radiation emission, this process does not alter the intrinsic properties of graphene [38] . Second, because graphene is inert to most of the molecules present in the CSE, such as H 2 , CO, C 2 H 2 . We have performed exactly the same experiment using H 2 instead of atomic H and no etching (not even molecular hydrogen adsorption) takes place. We have obtained exactly the same STM images as for the clean SiC surface ( Fig. 2a ). This accurate methodology allows us to test the influence of many parameters in the process. Our simulation experiments and calculations indicate that the size of the resulting PAHs strongly depends on the hydrogen concentration and the formation temperature. If atomic hydrogen is included in the system and temperature is much lower than 900 K, we just have adsorption of H on the surface. If the temperature exceeds 1,500 K, we have new graphene formation at the surface as it is etched away (the surface regenerates). To have efficient graphene erosion, temperature in the 900–1,200 K range and high doses of atomic hydrogen are required. Thus, in our experiment performed in UHV chambers, we have been able to mimic the most important conditions for SiC dust grains in the CSE, and this kind of research opens the door to use UHV-model systems to understand the precise role of co-absorption of molecules, other than hydrogen, and radiation in dust-processing mechanisms (for further understanding of the UHV equivalence of the CSE, see Supplementary Note 1 ). SiC is produced close to the evolved star as small-sized nanoparticles (typically few nm) and it has been proven that the crystallization rates of SiC grains can be very fast (≈μm h −1 ) at high temperatures [18] . In our experiment, we have used single-crystal surfaces to simulate the process, and one might think that the surface chemical properties of large extended crystals and nanoparticles could be completely different. However, this is not the case. Just a few crystallographic unit cells are required for recovering the bulk electronic structure of SiC. There are several high-resolution transmission electron microscopic studies using SiC nanoparticles of diameter about 5 nm revealing that the graphitization process takes place efficiently on high-temperature annealing [39] , [40] all around the SiC nanoparticle [22] . Therefore, our single-crystal approach can be seen as a suitable atomic scale description of the astrochemical processes taking place on the surface of both, micrometre- and nanometre-sized, SiC grains populating the CSE. The usual size of PAHs in the ISM is estimated to be in the range of hundreds of C atoms, in good agreement with the one that we have indentified in Fig. 2d , which has around 180 C atoms. Although Fig. 3d might give the erroneous impression that only small PAHs can be produced, we would like to remark that the PAH formed by our proposed mechanism can be quite large. This misleading idea is due to the reduced number of atoms that can be handled into the complex ab initio MD calculations we have performed. Moreover, one might think that in our model, the etching process will last forever cracking the formed PAHs into smaller and smaller pieces as time goes on. There are several factors promoting a self-stopping of the etching of graphene into PAHs. The efficiency of the process is strongly dependent on the underlying interface, as it is shown in the DFT calculated movies (see Supplementary Movies 3, 6 and 9 ). In other words, the graphene etching takes place efficiently because it is supported on a SiC grain. Once the PAH is decoupled from the SiC, etching is not an efficient mechanism. The hydrogen concentration and the temperature decrease as the PAH travel outwards in the CSE. PAHs arrive to regions of ISM where the H concentration can be considered negligible. The same occurs with the temperature, which rapidly decrease below 900 K. We have recorded STM images of H deposited on graphene at 300 K where H clusters are spotted on top of C atoms. This H adsorption process is also known to occur on PAHs and it is called hyperhydrogenation. We have not seen any adsorption or erosion when H 2 is used. Also, the smaller PAHs have less probability of interacting with the atomic hydrogen and a higher hydrogen adsorption energy. DFT calculations show that as you decrease the size of the PAH, the atomic hydrogen capture probability decreases. In this sense, there are two factors influencing the self-stopping hydrogenation of small PAHs. First, the size of the absorption area; the smaller the PAH, the lower the probability of scattering with an impinging adsorbate. Second, energetic considerations; the smaller a PAH, the higher the adsorption energy for an extra hydrogen (see Supplementary Note 4 and Supplementary Fig. 4 ). Therefore, graphene etching in the CSE is a self-limiting process yielding to significantly large PAHs. Finally, based on these experiments, we should not expect the formed ISM PAHs to have the identifiable structures. Mixtures of PAHs, aromatic-aliphatic molecules and hyperhydrogenated PAHs molecules have been proposed to account for the astronomical infrared observations [41] . All these aromatic chemical species can be produced out of the above-presented processing mechanism of the SiC dust. We are aware that in our experiments we observe the surface of the SiC grains instead of the produced PAHs. However, the latter is difficult as a priori our mechanism does not favour a particular size of the produced species, and a global increase in mass detection experiments can just be expected. In conclusion, we propose an alternative PAH top-down formation mechanism through graphene etching on the surface of SiC dust grains at ISM. This model is supported by a combination of different state-of-the-art experimental techniques with advanced computational methods. The good match between the available astrochemical information and the advanced surface science experimental methodology suggests that the problems of the former can be successfully understood through the techniques of the latter and opens the door to the investigation and modelling of other processes related to dust particles in ISM. Scanning tunnelling microscope STM experiments were performed in a UHV system with a base pressure 1 × 10 −10 mbar using an Omicron variable temperature scanning tunnelling microscope, which enables us to perform measurements while keeping the sample in the 40–300 K range. Tungsten tips were used to acquire topography images in constant current mode. The chamber is equipped with an atomic H flux source that produces hydrogen by H 2 thermal cracking (99% efficiency, no protons). The gas passes through a tungsten capillary kept at 2,500 K by electron bombardment. The sample was placed at 150 mm from the capillary. The chamber contains an annealing stage that heats the sample through direct heating. After hydrogen deposition with the SiC sample at high temperature, it is transferred to the STM for local measurements. Photoemission experiments Synchrotron radiation XPS measurements were performed at the SuperESCA beamline of Elettra, the third-generation synchrotron light source in Italy. Here the top-up mode of operation of the storage ring generating synchrotron radiation provides a stable photon flux in a wide range of photon energies. The end station of SuperESCA consists of an UHV chamber with base pressure of 1 × 10 −10 mbar. It is specifically designed for high-flux and high-resolution core level spectroscopy, particularly of adsorbates on single-crystal surfaces using soft X-ray synchrotron radiation. The atomic H doser of the STM apparatus was mounted in the chamber. The main chamber is equipped with a hemispherical electron analyser using an home-made delay line electron detection system. The overall energy resolution, comprising the analyser and the photon beam resolution, was better than 50 meV. C1 s core level peak decomposition into curve components The XPS spectra analysis of the results obtained at the SuperESCA beamline was performed using the FITT program after a Shirley background subtraction. The high resolution of the experimental system permits us to decompose the peaks into its basic curve components; every component reflects a particular electronic environment (that is, bonding configuration) and results from the convolution of a purely quantum Lorentzian energy distribution (full width at half maximum, 0.12–0.2 eV) with a Gaussian distribution (full width at half maximum, 0.4–0.7 eV) [42] . However, the carbon chemistry is very rich and the interpretation of the C1 s spectra is not straightforward. The components corresponding to sp 2 - and sp 3 -bonding configurations measured for pure graphite and pure diamond, respectively, appear at very similar binding energies (284.68 and 285.0 eV, respectively) [43] , [44] . We have decomposed the C1 s XPS peak of the as-grown G/SiC sample ( Fig. 4 ) in five different basic components without using any asymmetry parameter. SiC is a wide-gap semiconductor and therefore we use symmetrical peaks for the fitting. In Supplementary Fig. 1 , we show the C1 s and Si2 p photoelectron peaks decomposed in its basic components before and after H treatment. The component appearing at 284.83 eV can be directly assigned to the graphene contribution (or C atoms in sp 2 configuration), and is the biggest contribution to the C1 s core level peak, with its 58.2% of the total area. This component is also important for calibration of the energy width, since it is narrow enough to test the Lorentzian and Gaussian widths with a high precision. The components located at lower binding energies than the main peak (in our case 283.98 eV) are attributed normally to carbides, and we assign them to the C in the SiC bulk crystal [35] , [36] . There are three other components at higher binding energies, which can in principle be assigned to different configurations of C atoms in the superficial rearrangement that takes place on surface reconstruction [35] . We assign these XPS components to surface-related peaks and name them with an S. in the way that follows: S. C-Si 1 at 285.26 eV, S. C-Si 2 at 285.73 eV and S. C-Si 3 at 286.4 eV, respectively. We will later discuss the validity of this assumption. Theoretical spatially distributed density of states The molecular orbitals of the isolated PAHs have been calculated using the DFT calculation package FIREBALL. To resemble the experimental STM images of free PAHs, they have been taken as spatially distributed orbital densities, density of states, with suitable values of the orbital density three-dimensional isosurfaces to mimic the experimental morphology. Molecular dynamics The atomistic MD simulations have been performed by using the fast and efficient local-orbital DFT code FIREBALL. The temperature in these calculations is simulated by giving to each non-fixed atom a random initial velocity. In particular, to mimic the physical conditions for the etching of the graphene by atomic hydrogen, the dynamical processes were simulated giving to all the systems an initial temperature T =1,000 K. Then, the atoms were free to move using free MD up to a total time of 250 fs, corresponding to 250 MD steps. Three different graphenic configurations have been simulated by molecular dynamics: (a) two parallel 6 × 6 H-saturated flat graphene nanoribbons (with 132 atoms each) distanced by 3.35 Å; (b) the same two parallel 6 × 6 H-saturated flat graphene nanoribbons (with 132 atoms each) distanced by 3.35 Å as in previous case (a), but this time by including around 0.5 ML atomic hydrogen content in between the interlayer region, which initially forms an homogenous atomic H-intercalated layer; and, finally, (c) a 6 × 6 H-saturated flat graphene nanoribbon on a (fix) fully pre-optimized 6 × 6 fragment of a H-saturated on-SiC graphene buffer layer (at a distance of 3.35 Å), with the same interlayer atomic H content than in previous case (b). Atomic hydrogen adsorption potential energy curves The adsorption energy curves of atomic hydrogen in interaction with PAHs of different sizes have been obtained by using the accurate planewave DFT parametrization included in the QUANTUM ESPRESSO simulation package. In addition, to properly account the non-negligible dispersion forces appearing within this kind of interactions, we have used the DFT+D approach also implemented in the mentioned planewave simulation code. For this purpose, we have used a generalized gradient-corrected approximation for the electronic exchange-correlation description, and an empirical efficient van der Waals R −6 correction to add dispersive forces to conventional density functionals (DFT-D). Two different adsorption configurations have been analysed in the calculations: chemisorption and physisorption paths of atomic hydrogen approaching towards an ‘on-top’ PAH carbon atom adsorption site. How to cite this article: Merino, P. et al. Graphene etching on SiC grains as a path to interstellar polycyclic aromatic hydrocarbons formation. Nat. Commun. 5:3054 doi: 10.1038/ncomms4054 (2014).